Dual role of myosin II duringDrosophilaimaginal disc metamorphosis The motor protein non-muscle myosin II is a major driver of the movements that sculpt three-dimensional organs from two-dimensional epithelia. The machinery of morphogenesis is well established but the logic of its control remains unclear in complex organs. Here we use live imaging and ex vivo culture to report a dual role of myosin II in regulating the development of the Drosophila wing. First, myosin II drives the contraction of a ring of cells that surround the squamous peripodial epithelium, providing the force to fold the whole disc through about 90°. Second, myosin II is needed to allow the squamous cells to expand and then retract at the end of eversion. The combination of genetics and live imaging allows us to describe and understand the tissue dynamics, and the logic of force generation needed to transform a relatively simple imaginal disc into a more complex and three-dimensional adult wing. Animal organs develop primarily from simple epithelial sheets—tightly joined cells with apico–basal polarity but otherwise lacking three-dimensional structure. Patterning in the plane of the epithelium occurs when cells remodel contacts with their neighbours, either individually or in groups. These changes can lead, for example, to the differentiation of an organized epithelial mosaic of specialized cell types, as in the case of the Drosophila retina, or changes in the size and shape of the epithelium, as occurs in Drosophila germ band elongation [1] , [2] , [3] . Patterning in the third dimension, however, is less well characterized: how are two-dimensional epithelia transformed into the complex architecture of functional three-dimensional organs? It is nevertheless clear that some of the same processes of remodelling single cells can produce substantial tissue shape change. Overall, however, there are few cases where there is clear understanding of three-dimensional organ morphogenesis. Non-muscle myosin II (myosin II) is a contractile protein that in many contexts is responsible for sculpting the actin cytoskeleton of cells, leading to developmental shape changes. Myosin II is a hexamer of three pairs of subunits. In Drosophila, the myosin II heavy chain is encoded by zipper ( zip ) [4] , the regulatory light chain by spaghetti squash ( sqh ) [5] , [6] and the essential light chain by Mlc-c. The regulation of myosin II activity generates cell shape changes. Phosphorylation of the regulatory light chain induces myosin II activation (reviewed in Tan et al . [7] ) by increasing its recruitment to the cell cortex. This activation in the cortical region initiates apical contraction of the cell, which leads to a change from a columnar shape to a ‘bottle’ shape, narrower at the apical region than basally. This deformation can occur in groups of cells, generating a change in overall epithelial shape. For example, during formation of the ventral furrow in the Drosophila embryo or the morphogenetic furrow of the eye imaginal disc, a line of cells co-ordinately constrict apically to form an indentation [1] , [8] , [9] , [10] , [11] , [12] , [13] , [14] . A similar process happens during morphogenesis of the vertebrate neural tube in mammals [13] , [15] , [16] . In the case of the formation of tubular organs, such as the tracheal system of Drosophila , the process starts with the myosin II-induced apical constriction of a circular group of cells [17] , [18] . Asymmetric accumulation of myosin in the apical surface of the cells (only in some cell vertices and not in others) is related to other kinds of morphogenetic events, including intercalation of cells during the convergent extension of the Drosophila embryonic germ band [2] , and rotation of the ommatidia precursors in the eye imaginal disc [1] . The models above describe a deformation in a broadly homogeneous epithelium, where all the cells are equivalent in shape and size, and have similar physical attributes such as rigidity or elasticity. More complex systems include a variety of cell characteristics. For example, in Drosophila embryonic dorsal closure two kinds of cell are involved: squamous and columnar. Improvements in imaging techniques have been used to show that closure of the epidermis over the amnioserosa is a complex movement contributed by the pulsating force generated by the amnioserosa and the contraction of an acto-myosin ring in the cells of the leading edge [19] , [20] , [21] . We have investigated the morphogenetic mechanisms of a yet more complex structure, a three-dimensional tissue. The transformation during metamorphosis of the Drosophila wing imaginal disc into the adult wing involves extensive remodelling. Imaginal discs are more complex structures than often described: a continuous epithelial sac formed by two layers of different morphology, the peripodial epithelium (PE), mainly composed of squamous cells, and the disc proper (DP), mainly composed of columnar cells. A third class, cuboidal cells, situated towards the edge of the wing disc, forms a transition zone between the columnar and squamous epithelia [22] , [23] , [24] . Interplay between the layers underlies the organ sculpting movements of metamorphosis [23] , [25] , [26] , [27] , [28] . Eversion involves two major steps: folding of the disc and the retraction of the peripodial membrane [29] . We developed a method of ex vivo culture of imaginal wing discs [29] and have focused our analysis on the folding of the wing disc. We have described the main processes involved in this example of morphogenesis: where the forces are generated, the response of the surrounding cells and the genetic mechanisms involved. Strikingly, we have discovered that morphogenesis depends on a dual myosin II role. First, it accumulates throughout the cytoplasm of a ring of cuboidal cells, transforming them into a multicellular ‘drawstring’ that induces folding of the PE; second, it provides the squamous cells with the ability and strength necessary to expand in response to the induced tension. Elevated myosin II levels in a stripe of cells When imaginal discs are fixed for immunohistochemical analysis, the morphology of the squamous PE is disrupted. We therefore analysed gene expression by live imaging of unfixed discs ( Fig. 1a ). For clarity, we will divide the PE cells into two subtypes, the stripe cells ( Fig. 1b green) and central cells ( Fig. 1b , blue). The central cells are typical squamous cells, polygonal, very flat, with a large surface area; ( Fig. 1f ) the stripe cells surround the central cells; they are typically referred to as cuboidal, or border cells, although their actual shape is fusiform, with a cubic section and the longer axis of the cells parallel to the compartment boundary ( Fig. 1h , green; Fig. 1g ). 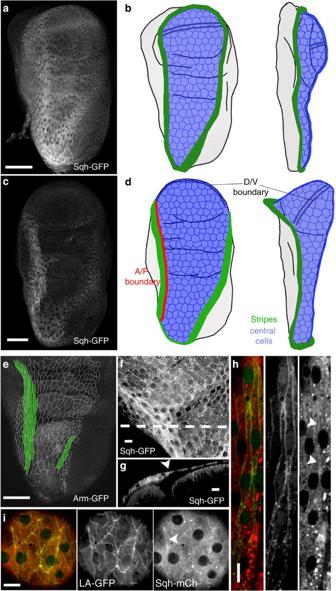Figure 1: Myosin II expression in the peripodial epithelium of the wing imaginal disc. (a) Sqh-GPF expression in a live third instar wing imaginal disc in sqh null mutant background. (b) Scheme showing relevant domains of the peripodial epithelium in a frontal (left) and a lateral (right) view at the same stage. The green regions are the stripes of cuboidal cells with the highest expression of myosin II. The blue region corresponds to the squamous central cells. (c) Sqh-GPF expression in a live prepupal wing disc in sqh null mutant background. Folds in the discs and a double line representing the D/V boundary are also shown in all the cartoons. (d) Scheme showing the stripes (green) and the central cells (blue) at late third instar stage. One of the stripes runs along the A/P boundary (red line) of the peripodial epithelium. (e) Cell outlines of the central and stripe cells traced from different confocal planes of an Arm-GFP unfixed wing disc. The stripe cells (green) are elongated parallel to the A/P axis. (f) Magnification of a Sqh-GFP disc at the border between stripe and central cells, near the hinge region. (g) Saggital view of the same disc at the position of the dotted line inf. The central PE cells are flatter than the stripe cells (white arrowhead marks the border between the cell types). High-resolution view of the expression of myosin II (red, Sqh-mCherry) and actin (green) in the stripe cells (h), labelled withodd-G4>UAS-lifeact-GFP, and the central cells (i), labelled withSqh-mCherry/Gug-G4>UAS-lifeact-GFP. Arrowheads in right side ofiandhshow regions of higher accumulation of myosin II, which co-localize with lifeact expression. Note that sqh-mcherry forms aggregates′ seen as bright puncta that are artefacts of the fluorescence protein. Scale bars, 50 μm (a,c,e); 10 μm (f,g,h,i). Figure 1: Myosin II expression in the peripodial epithelium of the wing imaginal disc. ( a ) Sqh-GPF expression in a live third instar wing imaginal disc in sqh null mutant background. ( b ) Scheme showing relevant domains of the peripodial epithelium in a frontal (left) and a lateral (right) view at the same stage. The green regions are the stripes of cuboidal cells with the highest expression of myosin II. The blue region corresponds to the squamous central cells. ( c ) Sqh-GPF expression in a live prepupal wing disc in sqh null mutant background. Folds in the discs and a double line representing the D/V boundary are also shown in all the cartoons. ( d ) Scheme showing the stripes (green) and the central cells (blue) at late third instar stage. One of the stripes runs along the A/P boundary (red line) of the peripodial epithelium. ( e ) Cell outlines of the central and stripe cells traced from different confocal planes of an Arm-GFP unfixed wing disc. The stripe cells (green) are elongated parallel to the A/P axis. ( f ) Magnification of a Sqh-GFP disc at the border between stripe and central cells, near the hinge region. ( g ) Saggital view of the same disc at the position of the dotted line in f . The central PE cells are flatter than the stripe cells (white arrowhead marks the border between the cell types). High-resolution view of the expression of myosin II (red, Sqh-mCherry) and actin (green) in the stripe cells ( h ), labelled with odd-G4 > UAS-lifeact-GFP , and the central cells ( i ), labelled with Sqh-mCherry / Gug-G4 > UAS-lifeact-GFP . Arrowheads in right side of i and h show regions of higher accumulation of myosin II, which co-localize with lifeact expression. Note that sqh-mcherry forms aggregates′ seen as bright puncta that are artefacts of the fluorescence protein. Scale bars, 50 μm ( a , c , e ); 10 μm ( f , g , h , i ). Full size image We found that the whole PE expressed high levels of myosin II, but that there was a pronounced increase in a stripe of cells that forms a ring of high expression. This stripe runs from the proximal tip of the disc, the stalk region, following a straight line along the A/P boundary, and then surrounds the cells of the wing pouch. The ring is finally closed with a more diffuse line of expression, along the posterior region over the notum ( Fig. 1a–d ). Interestingly, both stripe and central cells expressed high levels of Sqh-GFP (and Zip-GFP, not shown) at the interfaces between cells and throughout their cytoplasm. This contrasts with the columnar epithelium of the subjacent DP, where myosin was mainly accumulated in the apical region ( Fig. 1g ). As myosin II contractility works through its motor properties on actin fibres, we analyzed the distribution of F-actin in the PE cells using two different green fluorescent protein constructs, Lifeact-GFP and the actin binding domain of moesin [30] ( UAS-GMA-GFP , not shown). Both showed a similar accumulation pattern. Actin accumulated apically at the borders between central cells. This pattern is similar to the one found in the columnar cells at the DP. Interestingly, we also observed actin in prominent filamentous structures at the basal level of the cells ( Supplementary Fig. S1 ). The high levels of myosin II in the cytoplasm partially masks the co-localization with actin, but analysis of single confocal sections showed an enrichment of myosin II in the apical actin structures (arrowhead on Fig. 1i , right). The stripe cells also showed apical actin accumulation ( Fig. 1h ) that co-localized with slightly raised levels of myosin II (arrowheads on Fig. 1h , right). Like the PE cells, stripe cells showed basal accumulation of actin, forming fibre-like structures that run parallel to the long axis of the cells ( Supplementary Fig. S1 ). Behaviour of the central and stripe cells during eversion Comparing a mid third instar and a late third instar wing disc ( Fig. 1a ), it was apparent that the position of the myosin II stripe moved during development. The dorso–ventral boundary of the DP moves until it reaches the margin of the disc, allowing the apposition of dorsal and ventral surfaces of the wing (compare Fig. 1b ). This movement is accompanied by an expansion of the overlying PE, resulting in the ring of stripe cells being no longer visible in a frontal view of the pupal disc. In this view we could just see the lateral stripes, which themselves moved laterally as eversion proceeds ( Fig. 1a–d ; see also Fig. 6 for a schematic of the whole eversion process). To follow these changes in detail, we used real-time imaging to examine the movement of the PE during the first step of eversion, when the whole disc folds (about 3 h of ex vivo culture). As expected, we observed the displacement of the two stripes to the lateral region, eventually reaching the edges of the disc ( Fig. 2a , orange arrows; Supplementary Movie 1 ). A lateral view allowed us to follow the myosin II stripe parallel to the A/P boundary in its movement to the opposite face of the disc ( Fig. 2b ; Supplementary Movie 2 ). Three hours later, as the disc folded, the stripe cells ( Fig. 2b ) progressively moved and concentrated in a small region ( Fig. 2b , yellow arrow). This accumulation of cells with a high level of myosin II was also seen in unfixed discs dissected from the pupa at an equivalent stage to the cultured discs ( Fig. 2c ). The transition from a long stripe to a small cluster of cells suggested that the stripes were not only moving laterally, but also moved towards the stalk during this first phase of eversion—acting like a drawstring across the epithelium. To confirm our interpretation of this dynamic process, we tracked individual cells belonging to the A/P compartment boundary stripe, following how the nuclei displaced along the anterio–posterior border ( Fig. 2d ). In contrast to the movement of the stripe cells, central cells remained broadly static, showing that there is a net displacement of stripe cells with respect to the central cells ( Fig. 2d ; Supplementary Movie 3 ). The same was clear when comparing nuclei in the stripe, with nuclei in the adjacent row of central cells (white nuclei and blue nuclei, respectively, in Fig. 2e ; Supplementary Movie 4 ). 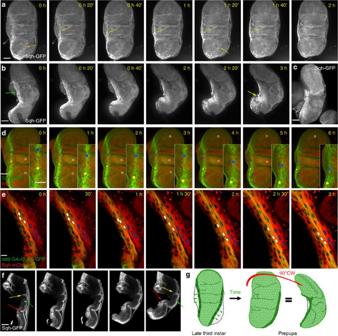Figure 2: Myosin II and the movements of the stripe cells during the eversion. (a) Frames fromSupplementary Movie 1: frontal view of a prepupal imaginal disc during the first steps of eversion. The disc is labelled with Sqh-GFP in a sqh null mutant background and shows the movement of the stripes (orange arrows). (b) Frames fromSupplementary Movie 2: lateral view of a Sqh-GFP imaginal disc in a sqh null mutant background. The stripe moves parallel to the A/P border (green arrow) towards a region at the lateral face (yellow arrow), from where later retraction of the PE will start. (c) A live Sqh-GFP wing imaginal disc dissected from an early pupa showing similar movement of the A/P stripein vivo. (d) Frames fromSupplementary Movie 3: the movement of stripe cells in a prepupal imaginal disc (green: Sqh-GFP; red, Histone2A-RFP). Dots track three individual cells and white circles label three central cells. The dots move towards the tip of the disc, while the circles stay relatively stationary. (e) Frames fromSupplementary Movie 4: the movement of stripe cells along the hinge lateral region. Stripe cells are labelled in green withodd-Gal4>UAS-lifeactin; myosin II labelled in red withSqh-mcherry. White dots mark three stripe cell nuclei which move relative to three cells outside the stripe marked with blue dots. (f) Section of a lateral view of a folding disc showing the movements of the disc proper. The middle fold (green arrow) disappears, the most proximal fold (red arrow) becomes deeper and the notum (yellow arrow) becomes more three-dimensional. (g) Stripe movements during the first steps of eversion. The PE stripe cells move proximally and laterally (black and green arrows, respectively). In the prepupa, the A/P stripe is not visible in a frontal view of the disc; in a lateral view (rotated 90° clockwise in the image), the highest accumulation of myosin II is concentrated in a shorter stripe at the lateral face of the now more three-dimensional disc. Note that in all figures time is approximate and time 0 corresponds to the starting point of image capture, not to a specific developmental stage. Scale bars, 50 μm (a,b,c,d,f); 10 μm (e). Figure 2: Myosin II and the movements of the stripe cells during the eversion. ( a ) Frames from Supplementary Movie 1 : frontal view of a prepupal imaginal disc during the first steps of eversion. The disc is labelled with Sqh-GFP in a sqh null mutant background and shows the movement of the stripes (orange arrows). ( b ) Frames from Supplementary Movie 2 : lateral view of a Sqh-GFP imaginal disc in a sqh null mutant background. The stripe moves parallel to the A/P border (green arrow) towards a region at the lateral face (yellow arrow), from where later retraction of the PE will start. ( c ) A live Sqh-GFP wing imaginal disc dissected from an early pupa showing similar movement of the A/P stripe in vivo . ( d ) Frames from Supplementary Movie 3 : the movement of stripe cells in a prepupal imaginal disc (green: Sqh-GFP; red, Histone2A-RFP). Dots track three individual cells and white circles label three central cells. The dots move towards the tip of the disc, while the circles stay relatively stationary. ( e ) Frames from Supplementary Movie 4 : the movement of stripe cells along the hinge lateral region. Stripe cells are labelled in green with odd-Gal4>UAS-lifeactin ; myosin II labelled in red with Sqh-mcherry . White dots mark three stripe cell nuclei which move relative to three cells outside the stripe marked with blue dots. ( f ) Section of a lateral view of a folding disc showing the movements of the disc proper. The middle fold (green arrow) disappears, the most proximal fold (red arrow) becomes deeper and the notum (yellow arrow) becomes more three-dimensional. ( g ) Stripe movements during the first steps of eversion. The PE stripe cells move proximally and laterally (black and green arrows, respectively). In the prepupa, the A/P stripe is not visible in a frontal view of the disc; in a lateral view (rotated 90° clockwise in the image), the highest accumulation of myosin II is concentrated in a shorter stripe at the lateral face of the now more three-dimensional disc. Note that in all figures time is approximate and time 0 corresponds to the starting point of image capture, not to a specific developmental stage. Scale bars, 50 μm ( a , b , c , d , f ); 10 μm ( e ). Full size image The above results imply that to accommodate stripe movement, there is a growth of the central territory of the PE. We have never observed any cell division in the PE at the stages of relevance to this work, so this expansion is most easily explained by enlargement of the surface area of the central squamous cells. We quantified this expansion by measuring the area stained by Grunge-Gal4, a marker of the central territory, of different discs at two stages, 0 h and 3.5 h of culture ( n =10 for each time point). We quantified what proportion of the whole disc surface is covered by Grunge-Gal4 expression: it increased from 64.4±6 to 87.0±8% (Student’s t -test P <0.00001, n =10 in each time point). The columnar epithelium of the DP also moved during these morphogenetic events. Specifically, the hinge region comprised three folds that can accommodate the bending of the wing disc. During the transition from the late third instar, when the wing disc is flat, to the more three-dimensional and folded stage, the middle fold ( Fig. 2f , green arrow) disappeared, while the proximal fold became deeper ( Fig. 2f , red arrow). At the same time, the notum adopted a more complex three-dimensional shape ( Fig. 2f ), and the wing continued protruding, to appose fully the dorsal and ventral compartments. Together, these observations present an overall morphogenetic scenario of the folding of the disc during the first phase of eversion. The dynamic distribution of myosin II enriched cells in the PE suggests that orchestrated myosin II-driven movement of the stripe cells could drive these large-scale tissue movements ( Fig. 2g ). Myosin II in the stripe is necessary to induce folding The cell dynamics and myosin II expression described above suggest that the ring of stripe cells could be a force generator that stretches the PE, thereby driving disc folding. On the other hand, the unusual distribution of myosin II throughout the cells, rather than just apically, makes them distinct from previously described cases where apical myosin II contractility controls morphogenesis. We directly tested the role of myosin II by examining the consequences of its reduction in the stripe cells ( Fig. 3a–d ; Supplementary Movies 1 and 5 ). To do this, we expressed specific RNA interference (RNAi) constructs against the myosin II heavy chain, zip , and the regulatory light chain, sqh , under the control of odd-Gal4 , a driver restricted in wing discs to the stripe cells ( Supplementary Fig. S2 ; Supplementary Movie 5 ). Expression of UAS-zip-RNAi effectively reduced the levels of Sqh-GFP (not shown), confirming its ability to reduce myosin II function. Knockdown of zip and sqh by RNAi caused comparable phenotypes (data not shown), although the effect of UAS-zip-RNAi was slightly stronger. 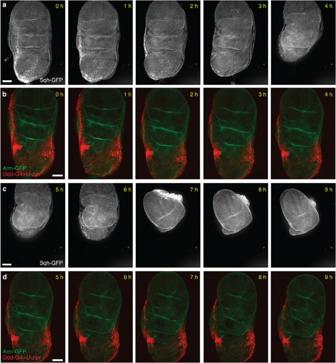Figure 3: Effect of the loss of function of myosin II in the stripes cells. (a,c) Frames fromSupplementary Movie 1showing the complete process of eversion including folding and the retraction. (b,d) Frames fromSupplementary Movie 5showing an Arm-GFP (green) disc where myosin II function has been reduced in the stripes (odd-Gal4>UAS-zip-RNAi,red). The stripes do not move laterally as they do in the control. The whole disc is it not able to fold properly, although the disc proper continues the normal morphological changes such as the apposition of wing dorsal and ventral compartments, and the deep increase of some folds. Scale bars, 50 μm. Figure 3: Effect of the loss of function of myosin II in the stripes cells. ( a , c ) Frames from Supplementary Movie 1 showing the complete process of eversion including folding and the retraction. ( b , d ) Frames from Supplementary Movie 5 showing an Arm-GFP (green) disc where myosin II function has been reduced in the stripes ( odd-Gal4 > UAS-zip-RNAi, red). The stripes do not move laterally as they do in the control. The whole disc is it not able to fold properly, although the disc proper continues the normal morphological changes such as the apposition of wing dorsal and ventral compartments, and the deep increase of some folds. Scale bars, 50 μm. Full size image Reduction of myosin II specifically in the stripe cells affected the whole process of eversion ( Fig. 3 ). Initially the disc was relatively normal but there was no lateral displacement of the stripes, and the first step of eversion was impaired: the columnar epithelium failed to make the 90° fold observed in wild-type (WT) discs ( Fig. 3a–d ). We also observed a later phenotype in which the stalk that attaches the disc to the pupal wall did not open, and there was no retraction of the PE at the end of eversion. In some cases, after more than 10 h the PE ruptured, usually over the wing pouch, and the developing wing emerged through the tear (not shown).These observations are based on six different movies that show the same phenotype. They suggest that lack of myosin II in the stripe cells eliminated the force necessary to generate disc folding. If this interpretation is correct, it implies that the folding force is generated by the movement of the stripes, not by the expansion of the central cells. At later stages the PE failed to retract, leading to a loss of final eversion. Force from the stripe generates tension over central cells As described above, the squamous cell layer expands during the early stages of eversion to accommodate the movement of the dorso–ventral border, and then expands further during eversion. When the stretching force from the stripe cells is abolished, the expansion of the central region is reduced ( Fig. 3b and d ), suggesting that central expansion is a direct consequence of movement of the adjacent stripe cells. However, cellular membranes are not elastic, so the expansion must be accommodated by cell growth and/or shape changes. In theory, the central cells will reach a point of maximum expansion beyond which continued application of force is likely to cause the whole disc to fold. To test the hypothesis that the central cells are under tension, we used laser surgery to make small holes in the central region of the PE ( n =12). We observed that as soon as the epithelium was cut, the size of the hole increased dramatically ( Fig. 4a–c ), indicating that it was indeed under tension. In many cases the tear in the PE continued as eversion progressed, and this prevented normal disc folding ( Fig. 4d ; Supplementary Movie 6 ). The increase in the size of holes cut in late third instar wing discs (mean=33.2-fold, n =4) was greater than when cut in mid third instar (mean=5.3-fold, n =4, P =0.049), further supporting the role of the stripe cells in generating tension as development proceeds. Between late third instar (mean=33.2-fold, n =4) and prepupal discs (mean=57.8-fold, n =4), the extent of increase also grew significantly ( P =0.047) ( Fig. 4c ), again indicating increasing tension in the PE over this period. Note that in some cases of very small cuts, wound healing mechanisms were able to reclose the hole, leading to normal eversion (not shown). Overall, these laser surgical manipulations strongly support the hypothesis that the central cells are put under progressive tension by the movement of the stripe cells. 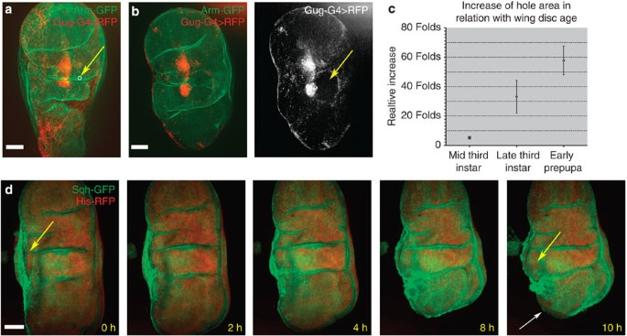Figure 4: Effect of laser ablation in the central cells during the eversion. (a) Late third instar disc before ablation (Arm-GFP, green; scattered central cells are labelled in red bygug-Gal4>UAS-RFP). The white circle indicated by the yellow arrow shows the size and location of the laser-cut hole. (b) The same disc 30 min after ablation. The hole (indicated by absence of red fluorescence, yellow arrow inb(right), has expanded dramatically). (c) Graph showing the fold increase of hole area over approximately 30 min versus age of the disc when the ablation was made.n=4 at each time point. Error bars represent s.d. (d) Frames fromSupplementary Movie 6showing a hole cut near to the A/P stripe (yellow arrow). After 2 h the wound healing process has reduced the area of the hole, but later the hole expands again and the folding of the whole disc is impaired. At 10 h the disc proper can be seen emerging from the hole; the opening of the stalk is also visible at this stage (white arrow). Scale bars, 50 μm. Figure 4: Effect of laser ablation in the central cells during the eversion. ( a ) Late third instar disc before ablation (Arm-GFP, green; scattered central cells are labelled in red by gug-Gal4 > UAS-RFP ). The white circle indicated by the yellow arrow shows the size and location of the laser-cut hole. ( b ) The same disc 30 min after ablation. The hole (indicated by absence of red fluorescence, yellow arrow in b (right), has expanded dramatically). ( c ) Graph showing the fold increase of hole area over approximately 30 min versus age of the disc when the ablation was made. n =4 at each time point. Error bars represent s.d. ( d ) Frames from Supplementary Movie 6 showing a hole cut near to the A/P stripe (yellow arrow). After 2 h the wound healing process has reduced the area of the hole, but later the hole expands again and the folding of the whole disc is impaired. At 10 h the disc proper can be seen emerging from the hole; the opening of the stalk is also visible at this stage (white arrow). Scale bars, 50 μm. Full size image Myosin II allows the expansion of the central cells Despite the central role for the stripe cells as force generators during epithelial folding, the central cells themselves also accumulated high levels of cytoplasmic myosin II. We investigated whether this was functionally important by knocking down myosin II with two different Gal4 drivers that are expressed in the central squamous cells: Grunge-Gal4 (Gug-Gal4) and Ubx LDN -Gal4 . As described above, Gug-Gal4 is not only expressed in the central squamous cells, but also in a few stripe cells and in the stalk (plus an additional expression in two patches of cells in the hinge region in the columnar epithelium) ( Fig. 5a and Aldaz et al . [29] ). Ubx LDN -Gal4 is patchily expressed only in cells of the squamous epithelium ( Supplementary Fig. S3 ). When zip or sqh were knocked down by Gug-Gal4 , elevated myosin II was still observed in stripes but the area occupied by the squamous cells at the late third instar/early prepupal stage was reduced. The cell number did not change, but the nuclei of these cells were more densely packed (compare Fig. 5e ), indicating that the area of individual cells was reduced. Unlike in WT discs, there was no increase of the central region over time when myosin II function was reduced by UAS-zip-RNAi overexpression (mean 56.1%±8 of apical area at time zero to 56.0%±7 at 3.5 h, n =10). This lack of expansion was most clear when comparing WT and myosin II knockdown discs after 3.5 h (central region 87.0%±8 of apical area in the WT background compared with 56.0% when myosin II was reduced; t -test, P <0.0001). These data suggest that myosin II is needed in the squamous cells to allow their expansion. 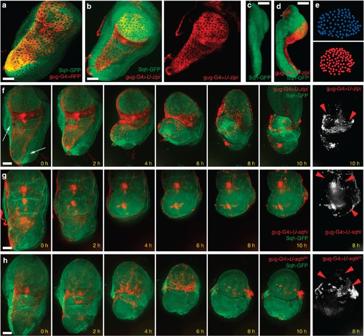Figure 5: Myosin II is required for the expansion of the central cells. (a) Prepupal disc;gug-Gal4>UAS-RFP(red) is expressed in central squamous cells; a few stripe cells (Sqh-GFP, green) also express gug-Gal4 (yellow). (b) A disc from the same stage where myosin II has been reduced in the central cells (gug-Gal4>UAS-zip-RNAi). The area of the red central cells is reduced. (c) Lateral view of a wild-type third instar wing disc showing that the peripodial epithelium covers the whole distal/proximal axis. (d) Lateral view of agug-Gal4>UAS-zip-RNAi/ UAS-RFP disc.The reduction of myosin II in the central cells causes misfolding of the disc; the wing pouch and notum are closer together. (e) Tracing of nuclei of the PM in the pouch region of the disc ina. (e) (bottom) Tracing of nuclei of the PM in the pouch region of the disc inb. (f) Frames fromSupplementary Movie 7of a disc where myosin II (green) has been strongly reduced (gug-Gal4>UAS-zip-RNAi) in the central cells of the PE (red). The white arrow indicates the remaining stripes. The disc folds in the opposite direction to normal (that is, the top surfaces of the notum and wing pouch move together). In the 8-h frame, the wing pouch is seen to rupture the central cells of the PE; the remaining central cells stay attached to the disc proper (red arrowheads). (g) Frames fromSupplementary Movie 8, where myosin II expression has been moderately reduced (gug-Gal4>UAS-sqh-RNAi). The area covered by the central cells (red) is similar to WT and the disc folds correctly, but retraction does not occur and several holes appear in the final frames (red arrowheads). (h) Frames fromSupplementary Movie 10showing agug-Gal4>UAS-sqhDD/UAS-RFPdisc. Strong activation of myosin II in the central cells (red) reduces their area. The disc proper shows some extra folds in the 0 h frame. The disc folds in the opposite way to WT, similar to the example ine. The retraction is aberrant and multiple holes are formed in the PE (red arrowheads). Scale bars, 50 μm. Figure 5: Myosin II is required for the expansion of the central cells. ( a ) Prepupal disc; gug-Gal4>UAS-RFP (red) is expressed in central squamous cells; a few stripe cells (Sqh-GFP, green) also express gug-Gal4 (yellow). ( b ) A disc from the same stage where myosin II has been reduced in the central cells ( gug-Gal4 > UAS-zip-RNAi ). The area of the red central cells is reduced. ( c ) Lateral view of a wild-type third instar wing disc showing that the peripodial epithelium covers the whole distal/proximal axis. ( d ) Lateral view of a gug-Gal4 > UAS-zip-RNAi/ UAS-RFP disc. The reduction of myosin II in the central cells causes misfolding of the disc; the wing pouch and notum are closer together. ( e ) Tracing of nuclei of the PM in the pouch region of the disc in a . ( e ) (bottom) Tracing of nuclei of the PM in the pouch region of the disc in b . ( f ) Frames from Supplementary Movie 7 of a disc where myosin II (green) has been strongly reduced ( gug-Gal4 > UAS-zip-RNAi ) in the central cells of the PE (red). The white arrow indicates the remaining stripes. The disc folds in the opposite direction to normal (that is, the top surfaces of the notum and wing pouch move together). In the 8-h frame, the wing pouch is seen to rupture the central cells of the PE; the remaining central cells stay attached to the disc proper (red arrowheads). ( g ) Frames from Supplementary Movie 8 , where myosin II expression has been moderately reduced ( gug-Gal4 > UAS-sqh-RNAi ). The area covered by the central cells (red) is similar to WT and the disc folds correctly, but retraction does not occur and several holes appear in the final frames (red arrowheads). ( h ) Frames from Supplementary Movie 10 showing a gug-Gal4 > UAS-sqh DD /UAS-RFP disc. Strong activation of myosin II in the central cells (red) reduces their area. The disc proper shows some extra folds in the 0 h frame. The disc folds in the opposite way to WT, similar to the example in e . The retraction is aberrant and multiple holes are formed in the PE (red arrowheads). Scale bars, 50 μm. Full size image In addition, a lateral view of the discs with reduced myosin II showed abnormal apposition between the wing pouch and notum region ( Fig. 5c ). Later defects included abnormal folds in the hinge area and, in some cases, unusual folding caused by the wing margin not reaching the border of the disc, and defective lateral displacement of the stripe cells. ( Fig. 5f , white arrow; Supplementary Movie 7 ). Stripe cells not expressing the Gug-Gal4 driver, and therefore unaffected by the myosin II knockdown, still moved, but because the stripes had not displaced laterally first, this caused the folding of the wing disc in the opposite direction to WT ( Fig. 5f ). This latter result supports the use of Gug-Gal4 driver for the study of the behaviour of central cells, as although some stripe cells are affected (and therefore have reduced myosin II activity) the remaining stripe cells can evidently still generate force as they are able to drive disc folding. At later stages, when myosin II was reduced, the retraction of the PE was impaired, the stalk did not open and PE retraction did not occur. Despite this disruption to the PE, the columnar DP epithelium developed relatively normally, with the apposition of dorsal and ventral compartments of the wing pouch leading to rupturing of the squamous epithelium and eversion through the hole ( Fig. 5f , red arrowhead; results based on five movies all with same phenotype). Using a single copy of UAS-sqh-RNAi construct (weaker than UAS-zip-RNAi ), the stripes were able to move to the lateral sides of the wing imaginal disc and the folding process occurred as in WT ( Fig. 5g ; Supplementary Movie 8 ). However, PE retraction was impaired, and the central region was ruptured on eversion ( Fig. 5g , red arrowheads; results based on three movies all with the same phenotype). Similar results were obtained using Ubx-Gal4 LDN line: overexpression of UAS-zip-RNAi or UAS-sqh-RNAi induced correct bending and posterior breakage of the PE in the region of the wing pouch ( Supplementary Movie 9 , and not shown; results based on six movies all with same phenotype). The weaker and patchy expression Ubx-Gal4 LDN line in just some cells of the PE allowed expansion of the central territory, however, the reduction of myosin II levels in these cells led to multiple ruptures in the central region. Overexpression of UAS-sqh DD (a Sqh form that mimics constitutive phosphorylation and activation) in the central cells using the Gug-G4 driver, also induced abnormal development ( Fig. 5h ; Supplementary Movie 10 ). Before eversion, the folds in the hinge and wing columnar epithelia were more pronounced, and the squamous epithelial surface appeared reduced. Upon eversion, the stripes tended to move to the sides and contract, but the central region did not expand correspondingly, so the stripes did not reach the other side of the disc. As with Gug-G4>UAS-zip-RNAi , stripe contraction therefore caused folding in the opposite direction to normal. But our data suggest that the similar phenotypes have different causes: while the reduction of myosin II in the central territory prevented cells from expanding, cells with over-activated myosin II are actively contracting (based on four movies with the same phenotype). Overall, these data imply that, like the stripe cells, the activity and levels of myosin II in the central cells must be tightly regulated, but in these cells, its role is to allow, first expansion of squamous cells, and then to mediate PE retraction. Recently developed live imaging techniques [29] have allowed us to analyse for the first time the tissue dynamics that underlie Drosophila imaginal wing disc eversion, an attractive model of organogenesis. We have also dissected the requirement of myosin II function in the peripodial epithelium (PE) to drive these complex movements ( Fig. 6 ). Two important distinctions between this model and previously described morphogenetic processes in which myosin II participates are, firstly, the heterogeneity of the tissue, with three quite distinct cell populations (squamous, cuboidal and columnar) and, secondly, the sculpting in three dimensions that occurs upon eversion. Unlike in many of the more two-dimensional systems, wing disc morphogenesis is not explained by myosin II-driven apical constriction of cells. Instead, myosin II throughout the cytoplasm of both the fusiform stripe cells, and the squamous central cells of the PE, is needed in different contexts for movement (of stripe cells) and expansion (of squamous cells). 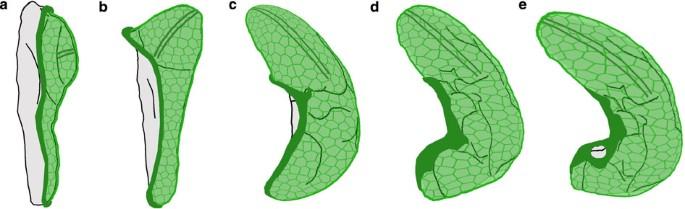Figure 6: Model of myosin II function during eversion. (a) In the third instar, the cuboidal stripe cells (dark green, indicating very high myosin II levels) surround the squamous central cells of the peripodial epithelium. (b) In the late third instar, the central cells (light green) start expanding to cover the larger surface created after the protrusion of the wing pouch. (c) The early prepupa develops a more three-dimensional wing disc. The contraction of the stripes together with the protrusion of the wing pouch induces the expansion of the central cells to cover the frontal and lateral faces of the wing disc, in addition to the large ventral surface of the wing. (d) The folding of the disc induced by the contraction of the myosin II stripes produces further expansion of the central cells. (e) The final stage of folding coincides with the start of the retraction, which starts at the stalk region, shown in grey near the bottom of the diagram. This is the moment of maximum expansion of the central cells and the maximum contraction of the stripes is reached. Figure 6: Model of myosin II function during eversion. ( a ) In the third instar, the cuboidal stripe cells (dark green, indicating very high myosin II levels) surround the squamous central cells of the peripodial epithelium. ( b ) In the late third instar, the central cells (light green) start expanding to cover the larger surface created after the protrusion of the wing pouch. ( c ) The early prepupa develops a more three-dimensional wing disc. The contraction of the stripes together with the protrusion of the wing pouch induces the expansion of the central cells to cover the frontal and lateral faces of the wing disc, in addition to the large ventral surface of the wing. ( d ) The folding of the disc induced by the contraction of the myosin II stripes produces further expansion of the central cells. ( e ) The final stage of folding coincides with the start of the retraction, which starts at the stalk region, shown in grey near the bottom of the diagram. This is the moment of maximum expansion of the central cells and the maximum contraction of the stripes is reached. Full size image We can now describe the epithelial events that cause eversion. First, the expansion of the central cells is necessary to accommodate the rotation of the dorso–ventral border of the disc proper (DP) [29] . This rotation situates the top of the stripe cells on the rear face of the wing disc. At the same time, the stripe cells flanking the central PE start moving. We show that this movement acts as a cellular drawstring that surrounds the presumptive wing. The tension thus induced leads to a further expansion of the squamous central cells, allowing the lateral displacement of the stripes around the edge of the disc, until they reach the opposite face, the point of maximum expansion. At this stage, further stripe movement causes folding. It is notable that our model requires contributions from all three cell types: initial pressure is generated by the columnar epithelium, which appears more rigid than the PE, and acts as a scaffold; the pulling force derives from the migration of the cuboidal stripe cells; and correct orientation of folding depends on the expansion of the squamous central cells. Although myosin II is well established as the primary motor of contraction that controls epithelial morphogenesis in many contexts, the role we have described in the stripe cells is distinct. In particular, although a purse-string mechanism has also been suggested during dorsal closure of the Drosophila embryo [19] , [31] , the cellular mechanisms underlying the generation of such contractile cables seem to be different in these two situations. During dorsal closure, myosin II contraction is limited to the apical part of the leading edge cells, while in wing disc stripe cells, myosin II accumulates throughout the whole cytoplasm. Instead of a large-scale reorganization of actin into long apical cables, as occurs in dorsal closure, migration of the cellular stripes in the wing disc is presumably mediated by the pre-existing network of F-actin in the cell. Interestingly, the myosin II-driven movements in the PE are coordinated with other movements in the proper epithelium, including the rotation or bending of the wing pouch that involves integrins and the recently described gene Dorsocross [32] , [33] . At the same time, we show that movement in the DP and PE are at least partially independent as the apposition of dorsal and ventral parts of the wing pouch occurred even when the PE retraction was impaired. In the central squamous cells of the PE, too, myosin II function appears unconventional. Strong reduction of myosin II prevents their expansion, while moderate reduction allows their expansion but weakens the squamous layer so that it is ruptured by the pressure generated by the pulling force from the stripes and the pushing from the underlying DP. In these cells, therefore, the role of myosin II is to confer flexibility and rigidity, allowing the squamous cells to expand in response to the force generated by neighbouring regions. This more passive function requires only moderate activation of myosin II, as hyperactivation (by overexpressing UAS-sqh DD ) makes the squamous cells contract, preventing their expansion. It has become clear over the last few years that the forces generated by non-muscle myosin and actin are major components of the machinery in a large number of contexts. However, within this broad spectrum of mechanisms, it is also clear that the logic of how myosin contractility is harnessed to shape tissues is quite diverse. As well as the previously established processes of cellular apical contraction, and the remodelling of neighbouring cell contacts within the plane of an epithelium, we can now add force generation by accumulation and activation of myosin in patterned groups of cells as a mode of controlling the architecture of tissue development. Fly stocks and genetics Flies were grown under standard culture techniques. The following lines were used: UAS-zip-RNAi , UAS-sqh-RNAi (Vienna Drosophila RNAi stock centre), UAS-sqh DD (ref. 34 ), sqh Δx3 sqh-GFP [35] , sqh-mCherry [36] , UAS-lifeact [30] , UAS-GMA-GFP [37] , arm-GFP , UAS-mRFP , Histone2A-mRFP1 (Flybase), odd-Gal4 (ref. 38 ), Grunge-Gal4 (ref. 39 ), Ubx-Gal4 LDN (ref. 40 ). Overexpression using the Gal4/UAS system [41] was performed at 25°C. Ex vivo imaging Dissection and mounting of the wing imaginal disc was performed as in Aldaz et al . [29] All the process was performed at room temperature. We have used three different confocal systems: a Zeiss LSM510 on an upright microscope; a Zeiss LSM 710 on an inverted microscope; and a Perkin Elmer spinning disk UltraVIEWERS with an Orca ER CCD camera (Hamamatsu). Typically we took between 80–120 Z-sections at 1 μm interval every 20/50 min. The images were analyzed using Adobe Photoshop CS2, Image J, and Volocity (Improvision) software. Surface measurements UAS-RFP, Grunge-Gal4/sqh-GFP and UAS-RFP, Grunge-Gal4/UAS-zip-RNAi;sqh-GFP late third instar larval discs were dissected and mounted in culture medium and immediately imaged or cultivated for 3.5 h before confocal imaging. The total apical area and the area occupied by central cells was measured in each image using ImageJ software. The proportion of central cells over the total surface was calculated dividing the ‘area occupied by central cells’ by ‘total area’. At least 10 images were measured for each of the four different conditions. Mean and s.d. were calculated and statistical significance of the comparisons was analysed using a two tailed Student’s t -test. Laser microdisection The discs were dissected using a Zeiss PALM Laser microdissection system. Discs were mounted in eversion media in an observation chamber [29] . Before dissection, a Z-stack of each disc was taken using a Perkin Elmer spinning disk microscope. Discs were dissected using the following settings: speed 30 mm s −1 , cut energy 60, cut focus 75. The parameters were experimentally determined to cut the PE without scarring or photobleaching the DP. To measure the hole in the PE, a similar area in approximately the same region (over the hinge of the disc) was selected in every disc, and a photograph of the dissection area was taken before dissection. Approximately 20 min after dissection, a second Z-stack was taken. Images were analysed using Image J to measure the size of the dissection area and the area of the hole generated. Statistical analysis of the data was performed using the statistic tools from Microsoft Excel. How to cite this article: Aldaz, S. et al . Dual role of myosin II during Drosophila imaginal disc metamorphosis. Nat. Commun. 4:1761 doi: 10.1038/ncomms2763 (2013).